Two splice variants of the IDD14 transcription factor competitively form nonfunctional heterodimers which may regulate starch metabolism Alternative splicing of primary gene transcripts provides eukaryotic cells, with a critical scheme for enriching transcriptome and proteome diversity. Here we report that alternative splicing of the Arabidopsis INDERMINATE DOMAIN 14 ( IDD14 ) transcription factor gene generates a competitive inhibitor in regulating starch metabolism. An alternatively spliced IDD14 form (IDD14β), which is produced predominantly under cold conditions, lacks functional DNA-binding domain but is able to form heterodimers with the functional IDD14 form (IDD14α). IDD14α–IDD14β heterodimers have reduced binding activity to the promoter of Qua-Quine Starch ( QQS ) gene that regulates starch accumulation. Transgenic Arabidopsis plants overproducing IDD14α (35S: IDD14α ) exhibited retarded growth with pale green leaves as appeared on QQS -overexpressing plants. Notably, IDD14β overproduction rescued the 35S: IDD14α phenotypes. We propose that alternative splicing of the IDD14 gene generates a self-controlled regulatory loop that may modulate starch accumulation in response to cold. The regulation of transcription factors by dynamic formation of dimers and protein complexes is an important component of gene regulatory networks that provides a way of diversifying the affinity and specificity of protein–DNA interactions [1] . It also generates a wide variety of DNA-binding protein complexes from a limited number of transcription factors and regulatory proteins in eukaryotic genomes. An illustrative example is a feedback regulatory module provided by competitive inhibitors that form nonfunctional heterodimers with specific transcription factors. Several competitive inhibitors have been reported in both animals [2] and plants [3] , [4] . The inhibitor of DNA-binding (ID) proteins have sequence similarities to a subset of basic helix–loop–helix (bHLH) transcription factors that are involved in cell proliferation and differentiation in animals [2] . However, because these inhibitor proteins lack the basic region required for DNA binding, they prevent bHLH transcription factors from binding to DNA by forming heterodimers that possess reduced affinity for substrate DNA [2] . A few competitive inhibitors have been characterized in plants in recent years. Similar to the structural organization of the ID proteins, the Little Zipper (ZPR) proteins consisting of 67–105 residues possess leucine zipper motifs that have limited sequence similarities to class III homeodomain-leucine zipper (HD-ZIP III) transcription factors functioning in shoot apical meristem formation and lateral organ development in Arabidopsis [3] , [4] . Although the ZPR proteins lack DNA-binding domains, they are able to competitively interact with HD-ZIP III transcription factors to form nonfunctional heterodimers. The MINI ZINC FINGER (MIF) proteins consisting of ∼ 100 residues also function in a similar manner [5] . They have zinc finger (ZF) motifs that mediate protein–protein interactions. However, they lack other protein motifs normally present in the zinc finger-homeodomain (ZHD) transcription factors that regulate leaf development and floral architecture. It has been shown that the MIF1 protein reduces the DNA-binding affinity of the ZHD5 transcription factor by forming MIF1-ZHD5 heterodimers [6] . Although it has not been proven yet, the KIDARI (KDR) proteins have been suggested to act as a negative regulator of some bHLH transcription factors, such as LONG HYPOCOTYL IN FAR-RED1, in photomorphogenesis [7] . Alternative splicing is a biochemical process by which the exons of a primary gene transcript are reconstituted in multiple ways. It allows production of multiple proteins from a single gene, extending the proteomic and functional diversity in eukaryotes. However, in some cases, alternatively spliced isoforms apparently lack protein domains required for protein activities, obscuring the necessity of alternative splicing. For example, the Arabidopsis FCA gene encodes an RNA-binding protein that promotes flowering. The primary FCA gene transcript is alternatively spliced to yield four transcripts: α, β, γ and δ. Among the four transcripts, only the γ transcript is considered to encode the putative full-size FCA protein [8] . In this work, we found that alternative splicing of a transcription factor gene serves as an active way of controlling the full-size transcription factor by producing a competitive inhibitor. Through genome-wide searches for alternatively spliced transcription factors in Arabidopsis , we identified a gene encoding the INDERMINATE DOMAIN 14 (IDD14) transcription factor. Alternative splicing of the IDD14 gene was induced under cold conditions, producing a spliced isoform IDD14β that lacks a functional DNA-binding domain. The IDD14β isoform attenuated the activity of the full-size IDD14α transcription factor by competitively forming nonfunctional heterodimers. The IDD14α transcription factor regulates starch metabolism by binding directly to the promoter of the QQS gene. The IDD14β form prevented the IDD14α transcription factor from binding to the QQS gene promoter, providing a distinct role of alternative splicing in gene expression regulation. Alternative splicing of IDD14 gene Protein structural analysis of plant transcription factors and their alternatively spliced isoforms suggest that at least some of the alternatively spliced isoforms lacking functional DNA-binding domains could act as competitive inhibitors. Recent studies have shown that a few alternatively spliced isoforms of animal transcription factors possess dominant negative activities [9] , [10] , supporting this hypothesis. We compared transcription factor genes with alternatively spliced genes in Arabidopsis and rice deposited in public databases. The in silico analysis predicted that ∼ 340 transcription factor genes undergo alternative splicing ( Supplementary Data 1 ). Among these, we chose Arabidopsis IDD14 gene for further analysis, as an alternatively spliced IDD14 isoform fit the structural rules defined by known competitive inhibitors. Comparing the two IDD14 cDNA sequences (designated IDD14α and IDD14β ) with genomic sequence revealed that the first intron was retained in the IDD14β cDNA ( Fig. 1a ). Reverse transcription PCR (RT–PCR) using cDNA-specific primers detected both transcripts ( Fig. 1b ). Whereas IDD14α contains three copies of ZF motifs, IDD14β lacks the ZF1 motif ( Fig. 1c and Supplementary Fig. S1 ). 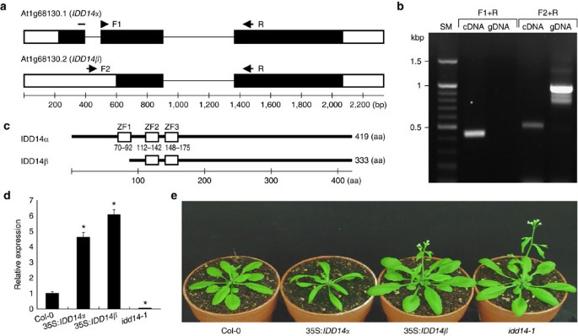Figure 1: Similar phenotypes of 35S:IDD14βtransgenic andidd14-1mutant plants. (a) Genomic structure ofIDD14and alternatively spliced variants. White boxes, untranslated regions; black boxes, exons; F1 and F2, forward primers; R, reverse primer. (b) Detection of alternatively spliced transcripts by RT–PCR and genomic PCR. SM, size marker. (c) Protein structure of IDD14 proteins. ZF, zinc finger. (d)IDD14gene expression. Transcript levels were determined by qRT–PCR using total RNA samples extracted from 2-week-old whole plants. Biological triplicates were averaged and statistically analysed using a Student'st-test (*P<0.01; 35S:IDD14α:P=0.0032,n=6; 35S:IDD14β:P=0.0002,n=6;idd14-1:P=0.0005,n=6). Bars indicate standard error of the mean. (e) Phenotypes of 35S:IDD14α, 35S:IDD14βandidd14-1plants. Figure 1: Similar phenotypes of 35S: IDD14β transgenic and idd14-1 mutant plants. ( a ) Genomic structure of IDD14 and alternatively spliced variants. White boxes, untranslated regions; black boxes, exons; F1 and F2, forward primers; R, reverse primer. ( b ) Detection of alternatively spliced transcripts by RT–PCR and genomic PCR. SM, size marker. ( c ) Protein structure of IDD14 proteins. ZF, zinc finger. ( d ) IDD14 gene expression. Transcript levels were determined by qRT–PCR using total RNA samples extracted from 2-week-old whole plants. Biological triplicates were averaged and statistically analysed using a Student's t -test (* P <0.01; 35S: IDD14α : P =0.0032, n =6; 35S: IDD14β : P =0.0002, n =6; idd14-1 : P =0.0005, n =6). Bars indicate standard error of the mean. ( e ) Phenotypes of 35S: IDD14α , 35S: IDD14β and idd14-1 plants. Full size image We produced transgenic plants overexpressing either the IDD14α or the IDD14β gene. We also obtained an IDD14 -deficient idd14 - 1 mutant ( Supplementary Fig. S2 ). The IDD14α -overexpressing plants exhibited retarded growth with pale green leaves showing some effects of gene dosage ( Supplementary Fig. S2 ). The 35S: IDD14α-3 transgenic line, which has a mild phenotype, was used in subsequent assays (hereafter referred to as 35S: IDD14α ). Whereas the levels of IDD14α and IDD14β transcripts were similar in the 35S: IDD14α and 35S: IDD14β transgenic plants, respectively ( Fig. 1d ), the 35S: IDD14β phenotypes were similar to those of the idd14-1 mutant in that both exhibited accelerated growth with slightly early flowering ( Fig. 1e and Supplementary Fig. S3 ). Attenuation of IDD14α activity by IDD14β We hypothesized that the 35S: IDD14β phenotypes would be due to the negative activity of IDD14β, possibly by forming heterodimers with IDD14α. IDD14α–IDD14β interactions were therefore examined in yeast cells, and, as expected, IDD14α and IDD14β formed heterodimers ( Fig. 2a ). In addition, as inferred from the structural organization, IDD14α and IDD14β formed homodimers. Assays using a series of IDD14α deletions revealed that the interactions occurred by the coiled-coil motif (residues 311–350; Fig. 2b ). In vitro pull-down assays using a recombinant maltose-binding protein-IDD14α (MBP-IDD14α) fusion and IDD14α and IDD14β proteins, which were produced by in vitro translation, confirmed that IDD14α forms homodimers ( Fig. 2c ) and heterodimers with IDD14β ( Fig. 2d ). Bimolecular fluorescence complementation (BiFC) assays in Arabidopsis protoplasts showed that IDD14α and IDD14β were co-localized into the nucleus ( Fig. 2e and Supplementary Fig. S4 ). We also obtained identical results from immunoprecipitation assays of protein extracts from Nicotiana benthamiana leaf cells expressing the MYC-IDD14α and MYC-IDD14β gene fusions ( Supplementary Fig. S5 ), further supporting the IDD14α–IDD14β interactions. 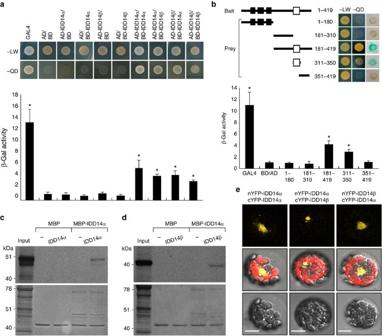Figure 2: IDD14α–IDD14β interactions. Inaandb, measurements of β-Gal activities were averaged and statistically treated (bottom panels). Bars indicate standard error of the mean. (a) Yeast coexpression assays. Cell growth on selective media without Leu, Trp, His and Ade (–QD) indicates positive interactions. β-Gal activities were normalized by dividing total activity by optical cell density (t-test, *P<0.01; GAL4:P=1.2×10−7,n=9; AD-IDD14α/BD-IDD14α:P=2×10−5,n=9; AD-IDD14α/BD-IDD14β:P=0.0012,n=9; AD-IDD14β/BD-IDD14α:P=1.8×10−4,n=9; AD-IDD14β/BD-IDD14β:P=0.0058,n=9). (b) Mapping of interacting domain. Interactions were examined both by cell growth on selective media (–QD) and by colony filter-lift assays (top panel;t-test, *P<0.01; GAL4:P=1.9×10−9,n=9; 181–419:P=0.0002,n=9; 311–350:P=0.0033,n=9). White box, coiled-coil motif. (c,d)In vitropull-down assays. A recombinant MBP-IDD14α fusion andin vitrotranslated radio-labelled IDD14α (c) and IDD14β (d) were used. Bottom panels were parts of Coomassie blue-stained gels. (e) BiFC assays. Partial YFP fusion constructs were transiently expressed inArabidopsisprotoplasts. Scale bar, 20 μm. Figure 2: IDD14α–IDD14β interactions. In a and b , measurements of β-Gal activities were averaged and statistically treated (bottom panels). Bars indicate standard error of the mean. ( a ) Yeast coexpression assays. Cell growth on selective media without Leu, Trp, His and Ade (–QD) indicates positive interactions. β-Gal activities were normalized by dividing total activity by optical cell density ( t -test, * P <0.01; GAL4: P =1.2×10 −7 , n =9; AD-IDD14α/BD-IDD14α: P =2×10 −5 , n =9; AD-IDD14α/BD-IDD14β: P =0.0012, n =9; AD-IDD14β/BD-IDD14α: P =1.8×10 −4 , n =9; AD-IDD14β/BD-IDD14β: P =0.0058, n =9). ( b ) Mapping of interacting domain. Interactions were examined both by cell growth on selective media (–QD) and by colony filter-lift assays (top panel; t -test, * P <0.01; GAL4: P =1.9×10 −9 , n =9; 181–419: P =0.0002, n =9; 311–350: P =0.0033, n =9). White box, coiled-coil motif. ( c , d ) In vitro pull-down assays. A recombinant MBP-IDD14α fusion and in vitro translated radio-labelled IDD14α ( c ) and IDD14β ( d ) were used. Bottom panels were parts of Coomassie blue-stained gels. ( e ) BiFC assays. Partial YFP fusion constructs were transiently expressed in Arabidopsis protoplasts. Scale bar, 20 μm. Full size image Our observations suggest that IDD14β would attenuate the DNA-binding activity of IDD14α homodimers by competitively forming heterodimers. To examine this, the IDD14β gene was expressed under the control of a methionine (Met)-suppressible promoter in yeast cells expressing BD-IDD14α and AD-IDD14α fusions. β-Galactosidase (β-Gal) activity assays showed that IDD14β induction substantially repressed the formation of IDD14α homodimers ( Fig. 3a–c ). To examine the negative activity of IDD14β in planta , we genetically crossed 35S: IDD14α plants with 35S: IDD14β plants. As inferred from the suppression of IDD14α homodimer formation by IDD14β, 35S: IDD14α phenotypes were rescued in the 35S: IDD14α X 35S: IDD14β plants ( Fig. 3d ), demonstrating that IDD14β negatively regulates IDD14α activity by inhibiting its homodimer formation. 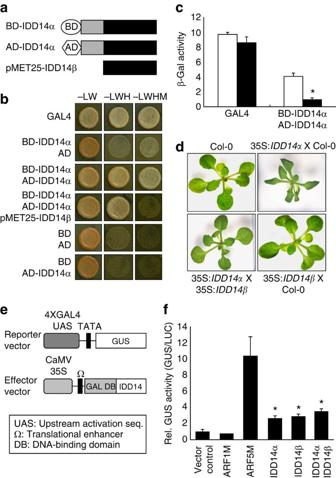Figure 3: Competitive inhibition of IDD14α activity by IDD14β. (a) Constructs used for yeast three-hybrid assays. TheIDD14βgene was expressed under the control of the methionine (Met)-suppressible promoter (pMET25-IDD14β). AD, activation domain; BD, DNA-binding domain. (b) Inhibition of IDD14α dimer formation by IDD14β. TheIDD14βgene is not expressed on selective media without Leu, Trp and His (–LWH), but expressed on selective media without Leu, Trp, His and Met (–LWHM). (c) Quantification of yeast coexpression assays. β-Gal activities were measured in the presence (white bars) or absence (black bars) of Met (t-test, *P=0.0013,n=12). (d) Suppression of 35S:IDD14αphenotypes byIDD14βcoexpression. (e) Reporter and effector vectors used for transient expression assays inArabidopsisprotoplasts. GAL4 transient expression assays were carried out as described previously11. TheRenillaluciferase gene served as an internal control to normalize values in individual assays. (f) Transcriptional activation activity of IDD14 isoforms. Five independent measurements were averaged. Bars indicate standard error of the mean (t-test, *P<0.01; IDD14α:P=0.0042,n=15; IDD14β:P=0.001,n=15; IDD14α IDD14β:P=3.2×10−6,n=15). Figure 3: Competitive inhibition of IDD14α activity by IDD14β. ( a ) Constructs used for yeast three-hybrid assays. The IDD14β gene was expressed under the control of the methionine (Met)-suppressible promoter (pMET25-IDD14β). AD, activation domain; BD, DNA-binding domain. ( b ) Inhibition of IDD14α dimer formation by IDD14β. The IDD14β gene is not expressed on selective media without Leu, Trp and His (–LWH), but expressed on selective media without Leu, Trp, His and Met (–LWHM). ( c ) Quantification of yeast coexpression assays. β-Gal activities were measured in the presence (white bars) or absence (black bars) of Met ( t -test, * P =0.0013, n =12). ( d ) Suppression of 35S: IDD14α phenotypes by IDD14β coexpression. ( e ) Reporter and effector vectors used for transient expression assays in Arabidopsis protoplasts. GAL4 transient expression assays were carried out as described previously [11] . The Renilla luciferase gene served as an internal control to normalize values in individual assays. ( f ) Transcriptional activation activity of IDD14 isoforms. Five independent measurements were averaged. Bars indicate standard error of the mean ( t -test, * P <0.01; IDD14α: P =0.0042, n =15; IDD14β: P =0.001, n =15; IDD14α IDD14β: P =3.2×10 −6 , n =15). Full size image However, the transcriptional activation activity of IDD14α was unaffected by IDD14β, as assayed by the transient expression assays in Arabidopsis protoplasts [11] ( Fig. 3e,f ), suggesting that the negative activity of IDD14β is due to the inhibition of DNA binding. Binding of IDD14α to the QQS gene promoter The 35S: IDD14α phenotypes, such as growth retardation and pale green leaves with downward curling ( Supplementary Fig. S2 ), are frequently observed in plants with disturbed sugar metabolism [12] , [13] , suggesting that the IDD14 gene may have metabolic roots. In support of this view, several IDD members have been implicated in sugar and starch metabolism in Arabidopsis and maize [14] , [15] . To better understand the physiological role of IDD14, we examined the expression of an extensive set of genes that are involved in sugar and starch metabolism in 35S: IDD14α and 35S: IDD14β transgenic and idd14-1 mutant plants. We found that only the QQS gene was significantly upregulated in 35S: IDD14α transgenic plants ( Fig. 4a and Supplementary Fig. S6 ). Notably, the QQS gene was downregulated in 35S: IDD14β transgenic plants, as occurred in idd14-1 mutant. However, QQS gene expression was recovered in the 35S: IDD14α ×35S: IDD14β plants, suggesting that IDD14α activity is correlated with the QQS gene. 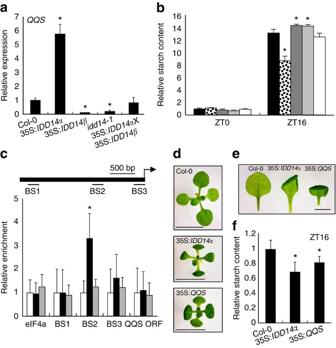Figure 4: Regulation of theQQSgene by IDD14 proteins. (a)QQSgene expression. Transcript levels were determined by qRT–PCR. Biological triplicates were averaged and statistically treated (t-test, *P<0.01; 35S:IDD14α:P=2.2×10−8,n=6; 35S:IDD14β:P=0.0001,n=6;idd14-1:P=5×10−5,n=6). Bars indicate standard error of the mean. (b) Measurements of starch contents. The value 1 is equal to 0.3 mg per g fresh weight. Bars indicate standard error of the mean. Black bars, Col-0; dotted bars, 35S:IDD14α; dark grey bars, 35S:IDD14β; light grey bars,idd14-1; white bars, 35S:IDD14α×35S:IDD14β(t-test, *P<0.01; 35S:IDD14α:P=1.2×10−6,n=12; 35S:IDD14β:P=0.005,n=12;idd14-1:P=0.0061,n=12). (c) Chromatin immunoprecipitation assays. BS1, BS2 and BS3 are putative binding sites in theQQSgene promoter (top panel). Three-week-old plants were used. Three measurements were averaged and statistically treated (bottom panel;t-test, *P=0.0076,n=9). Bars indicate standard error of the mean. White bars, Col-0; black bars, 35S:IDD14α-MYC; grey bars, 35S:IDD14β-MYC. (d) Phenotypes of 35S:IDD14αand 35S:QQStransgenic plants. Scale bar, 5 mm. (e) Leaf morphology. Scale bar, 2 mm. Indande, 10-day-old plants were photographed. (f) Starch contents of 35S:IDD14αand 35S:QQStransgenic plants. The value 1 is equal to 2.2 mg per g fresh weight. Bars indicate standard error of the mean (t-test, *P<0.01; 35S:IDD14α:P=1.6×10−6,n=18; 35S:QQS:P=0.002,n=18). Inbandf, five measurements were averaged and statistically analysed. Bars indicate standard error of the mean. ZT, zeitgeber time. Figure 4: Regulation of the QQS gene by IDD14 proteins. ( a ) QQS gene expression. Transcript levels were determined by qRT–PCR. Biological triplicates were averaged and statistically treated ( t -test, * P <0.01; 35S: IDD14α : P =2.2×10 −8 , n =6; 35S: IDD14β : P =0.0001, n =6; idd14-1 : P =5×10 −5 , n =6). Bars indicate standard error of the mean. ( b ) Measurements of starch contents. The value 1 is equal to 0.3 mg per g fresh weight. Bars indicate standard error of the mean. Black bars, Col-0; dotted bars, 35S: IDD14α ; dark grey bars, 35S: IDD14β ; light grey bars, idd14-1 ; white bars, 35S: IDD14α ×35S: IDD14β ( t -test, * P <0.01; 35S: IDD14α : P =1.2×10 −6 , n =12; 35S: IDD14β : P =0.005, n =12; idd14-1 : P =0.0061, n =12). ( c ) Chromatin immunoprecipitation assays. BS1, BS2 and BS3 are putative binding sites in the QQS gene promoter (top panel). Three-week-old plants were used. Three measurements were averaged and statistically treated (bottom panel; t -test, * P =0.0076, n =9). Bars indicate standard error of the mean. White bars, Col-0; black bars, 35S: IDD14α-MYC ; grey bars, 35S: IDD14β-MYC . ( d ) Phenotypes of 35S: IDD14α and 35S: QQS transgenic plants. Scale bar, 5 mm. ( e ) Leaf morphology. Scale bar, 2 mm. In d and e , 10-day-old plants were photographed. ( f ) Starch contents of 35S: IDD14α and 35S: QQS transgenic plants. The value 1 is equal to 2.2 mg per g fresh weight. Bars indicate standard error of the mean ( t -test, * P <0.01; 35S: IDD14α : P =1.6×10 −6 , n =18; 35S: QQS : P =0.002, n =18). In b and f , five measurements were averaged and statistically analysed. Bars indicate standard error of the mean. ZT, zeitgeber time. Full size image The QQS gene negatively regulates starch accumulation [16] . Measurements of starch content revealed that it was detectably lower in 35S: IDD14α transgenic plants ( Fig. 4b ). In contrast, it was elevated by ∼ 8% in 35S: IDD14β transgenic and idd14-1 mutant plants. Meanwhile, the starch content in 35S: IDD14α ×35S: IDD14β plants was similar to that in Col-0 plants, in agreement with QQS expression patterns. To rule out the possibility that differential starch contents are caused by developmental defects owing to the constitutive expression of IDD14 genes, we produced transgenic plants expressing IDD14α and IDD14β genes under a β-estradiol-inducible promoter and measured starch contents 3 days after induction. Whereas starch content was significantly reduced in IDD14α -expressing plants, it was largely uninfluenced in IDD14β -expressing plants ( Supplementary Fig. S7 ), supporting the linkage of the IDD14 transcription factor with starch accumulation and disturbed starch metabolism as the cause of the pale green appearance of 35S: IDD14α transgenic plants. To explore whether IDD14 transcription factors directly regulates the QQS gene, we fused a MYC-coding sequence in-frame to the 3′ ends of IDD14α and IDD14β genes and transformed the expression construct into Arabidopsis plants. Chromatin immunoprecipitation assays were performed using 35S: IDD14α-MYC and 35S: IDD14β-MYC transgenic plants. The results showed that IDD14α bound to the BS2 sequence that covers residues −924 to −637 in the QQS gene promoter ( Fig. 4c ). In contrast, no discernible binding activity was detected with IDD14β, showing that partial loss of the ZF domains in IDD14β disrupts its DNA-binding activity. The functional relationship between IDD14 and the QQS gene was also supported by phenotypic analysis. Both 35S: IDD14α and 35S: QQS transgenic plants showed similar phenotypes, such as retarded growth and downward leaf curling ( Fig 4d,e ), and low starch content ( Fig. 4f ). Furthermore, although starch content was higher in 35S: IDD14β transgenic plants, it was significantly reduced in the genetic cross of 35S: IDD14β and 35S: QQS transgenic plants ( Supplementary Fig. S8 ), confirming that QQS functions downstream of the IDD14α transcription factor. Cold-induced IDD14 alternative splicing in starch metabolism A critical question that remained was how IDD14 alternative splicing was induced. We examined the effects of growth hormones, sugars and various stresses on the relative ratio of IDD14α and IDD14β transcripts. Interestingly, IDD14 alternative splicing was greatly influenced only by cold (4 °C; Fig. 5a ). Whereas the level of IDD14α transcript was unchanged, the level of IDD14β transcript was gradually elevated in response to cold. In contrast, the level of QQS transcript steadily decreased, consistent with the notion that IDD14β negatively regulates the activity of IDD14α that activates the QQS gene. The QQS gene was not influenced by other environmental signals and sugars ( Supplementary Fig. S9 ). 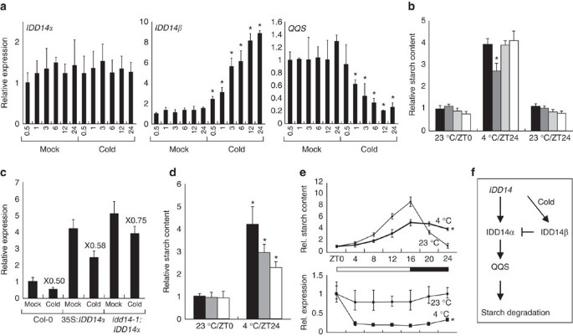Figure 5: Cold induction ofIDD14alternative splicing. (a) Effects of cold onIDD14andQQSgene expression (t-test, *P<0.01,n=6). Two-week-old plants were treated with cold. (b) Effects of cold on starch accumulation. Black bars, Col-0; dark grey bars, 35S:IDD14α; light grey bars, 35S:IDD14β; white bars,idd14-1(t-test, *P=0.0033,n=15). (c) Effects of cold onQQSgene expression. Two-week-old plants were treated with cold. (d) Measurements of starch contents. Black bars, Col-0; grey bars, 35S:IDD14α; white bars,idd14-1:IDD14α(t-test, *P<0.01; Col-0:P=3.1×10−8,n=15; 35S:IDD14α:P=0.0002,n=15;idd14-1:IDD14α:P=0.0015,n=15). Inbandd, cold treatment was initiated at ZT0. (e) Kinetic measurements of starch contents (top panel) andQQSgene expression (bottom panel). Plants at ZT0 were exposed to cold (t-test, *P<0.01,n=15). (f) Working model of the IDD14-mediated regulatory module in starch accumulation under cold conditions. Ina,cande, transcript levels were determined by qRT–PCR. Whole plants were used for total RNA extraction. Biological triplicates were averaged and statistically treated. Inb,dande, shoots of two-week-old plants grown on Murashige and Skoog agar plates were used for starch extraction. Five measurements were averaged and statistically treated. The value 1 is equal to 0.3 mg per g fresh weight. Figure 5: Cold induction of IDD14 alternative splicing. ( a ) Effects of cold on IDD14 and QQS gene expression ( t -test, * P <0.01, n =6). Two-week-old plants were treated with cold. ( b ) Effects of cold on starch accumulation. Black bars, Col-0; dark grey bars, 35S: IDD14α ; light grey bars, 35S: IDD14β ; white bars, idd14-1 ( t -test, * P =0.0033, n =15). ( c ) Effects of cold on QQS gene expression. Two-week-old plants were treated with cold. ( d ) Measurements of starch contents. Black bars, Col-0; grey bars, 35S: IDD14α ; white bars, idd14-1:IDD14α ( t -test, * P <0.01; Col-0: P =3.1×10 −8 , n =15; 35S: IDD14α : P =0.0002, n =15; idd14-1:IDD14α : P =0.0015, n =15). In b and d , cold treatment was initiated at ZT0. ( e ) Kinetic measurements of starch contents (top panel) and QQS gene expression (bottom panel). Plants at ZT0 were exposed to cold ( t -test, * P <0.01, n =15). ( f ) Working model of the IDD14-mediated regulatory module in starch accumulation under cold conditions. In a , c and e , transcript levels were determined by qRT–PCR. Whole plants were used for total RNA extraction. Biological triplicates were averaged and statistically treated. In b , d and e , shoots of two-week-old plants grown on Murashige and Skoog agar plates were used for starch extraction. Five measurements were averaged and statistically treated. The value 1 is equal to 0.3 mg per g fresh weight. Full size image We next examined the effects of cold on the accumulation of starch. Plants were exposed to cold at zeitgeber time 0 (ZT0), and relative starch contents were measured at ZT0 and ZT24. Starch contents were low at ZT0 and ZT24 in plants incubated at 23 °C ( Fig. 5b ), as has been reported previously [16] , [17] . Starch accumulated rapidly during the light period but degraded during the dark period. In contrast, under cold conditions, starch contents increased approximately fourfold in 35S: IDD14β transgenic and idd14-1 mutant plants as they did in Col-0 plants at ZT24, which is consistent with the suppression of the QQS gene by cold ( Supplementary Fig. S10 ). However, the degree of elevation was reduced in 35S: IDD14α transgenic plants, probably because of the increased QQS activity. These observations indicate that starch degradation is reduced during the dark period in response to cold. The effects of IDD14β on the expression of the QQS gene in response to cold was verified by examining levels of QQS transcript in 35S: IDD14α transgenic plants and in the idd14-1 mutant overexpressing the IDD14α gene ( idd14-1:IDD14α ). The level of QQS transcript was reduced by ∼ 45% in 35S: IDD14α transgenic plants as it was in Col-0 plants exposed to cold ( Fig. 5c ). However, it was reduced by 25% in idd14-1:IDD14α plants. These data are at least, in part, explained by the negative regulation of IDD14α activity by IDD14β. Measurements of starch contents also support the role of IDD14β on the expression of QQS gene in regulating starch accumulation. Starch contents were lower in idd14-1:IDD14α plants than in 35S: IDD14α transgenic plants under cold ( Fig. 5d ). To explore the biological meaning of the starch accumulation with regard to temperature, patterns of starch accumulation were monitored throughout the ZT times after exposure to cold. Starch still accumulated during the light period but to a lesser degree than in plants incubated at 23 °C ( Fig. 5e ). After ZT16, whereas starch content rapidly decreased in plants grown at 23 °C, it was only slightly reduced in plants exposed to cold, which is in agreement with the suppression of the QQS gene that occurs in plants under cold conditions ( Fig. 5e ). Together, these observations indicate that the regulation of the QQS gene by IDD14 alternative splicing is physiologically important during the dark period and when plants are exposed to cold ( Fig. 5f ). RNA splicing is a post-transcriptional event that excises intron sequences from primary RNA transcripts and serves as a gene regulatory step in many eukaryotic genes. Alternative splicing generates multiple mRNAs from a single genetic locus through alternative selection of splice sites in the primary RNA transcripts, extending structural and functional diversities from the limited number of genes in the genome [8] . Alternative splicing of transcription factor genes has rarely been documented in plants, mostly because of nonfunctionality of the truncated forms. In this work, we demonstrated that an alternative spliced IDD14 isoform (IDD14β) has a functional role in starch metabolism under cold conditions. The IDD14 transcription factor funcitons as homodimers in regulating target genes. The IDD14β isoform lacks functional DNA-binding domain and thus is unable to bind to DNA. However, as it possesses intact protein–protein interaction domain, it can form heterodimers with the functional IDD14α form. The heterodimers has reduced DNA-binding activity. Therefore, the IDD14β isoform is functionally very similar to the competitive peptide inhibitors, such as ZPR3 (refs 3 , 4 ). It is envisaged that competitive inhibition of transcription factors by truncated isoforms provides a versatile regulatory scheme in gene expression regulation under stress conditions. Subtle changes in the ratio of intact transcription factors and alternatively spliced variants would profoundly affect expression of target genes. It seems that alternative splicing, in coordination with gene transcriptional control, may help to maintain the appropriate level of transcription factor activities under a given growth conditions. Furthermore, it is also envisioned that alternative splicing of transcription factors guarantees prompt transcriptional responses to environmental fluctuations. Several more competitive peptide inhibitors, in addition to ZPR proteins, have been identified recently in plants as well as in animals. Interestingly, phylogenetic analyses of genes encoding the competitive inhibitors and their target transcription factors in representative land plants, suggest that they are derived from functional transcription factor by deletion of functional domains before diversification of seed plants [3] . For example, although ZHD transcription factors are conserved in many land plants, including angiosperms, gymnosperms, seedless vascular plant ( Selaginella ) and nonvascular plant (moss), their competitive inhibitors MIFs are found only in seed plants, such as Arabidopsis , rice and cotton, supporting the recent occurrence of competitive inhibitors [6] . Similarly, ZPR proteins are present in Arabidopsis , rice and maize, but not in other plant databases [3] . The IDD14 transcription factor is regulated by a competitive inhibitor that is produced by alternative splicing. Comparative genomic analysis showed that it is conserved in diverse plant species ( Supplementary Table S1 ). So far, alternative splicing of the IDD14 gene was demonstrated only in Arabidopsis and has been predicted in rice ( http://www.plantgdb.org ). It is likely that competitive inhibition of transcription factors by alternatively spliced variants has a recent evolutionary origin. Starch accumulation is closely linked to plant responses to cold stress. Soluble sugars accumulate during the light period under cold conditions, and controlled starch degradation has a role in this process [18] , [19] , [20] , [21] , [22] . Our data strongly support that alternative splicing of IDD14 modulates its role in regulating starch metabolism under cold conditions. The IDD14α form regulates directly the QQS gene that induces starch degradation [16] . The QQS gene is repressed by cold via the self-regulatory module provided by cold-induced alternative splicing of IDD14. On the basis of previous observations, as well as our own, we propose that the competitive inhibition of IDD14α activity by an alternatively spliced variant IDD14β would serve as a cold adaptation strategy, helping a plant maintain a certain amount of starch during the dark period; this starch may be required to withstand cold conditions during the light period. We found that QQS gene has a role in IDD14 regulation of starch metabolism in Arabidopsis , in which an alternatively spliced variant acts as a self-regulatory inhibitor. Molecular genetic analysis also supports the negative role of QQS gene in starch accumulation. However, it is premature to generalize our findings. No QQS gene homologues have been characterized in other plant species yet. Although the QQS gene acts as a negative regulator of starch accumulation [16] , it is unknown how it influences starch metabolism. More studies are required to see whether the IDD14 regulation of QQS gene is also applicable to other plant species. It will also be worthy to explore the biochemical role of QQS protein in regulating sugar metabolism. In addition, broader searches for the targets of IDD14 transcription factor, in addition to QQS , would be helpful in resolving the uncertainties. Plant materials and growth conditions All Arabidopsis thaliana lines used were in the Col-0 background. Plants were grown in a controlled culture room at 22 °C with a relative humidity of 55% under long days (16-h light/8-h dark) with white light illumination (120 μmol photons per m 2 s) provided by fluorescent FLR40D/A tubes (Osram). The idd14-1 mutant (GABI_655E05) was isolated from a mutant pool of T-DNA insertion lines deposited in the Nottingham Arabidopsis Stock Centre (University of Nottingham, UK). Homozygotic lines were obtained by herbicide selection for three or more generations and by analysis of segregation ratios. Analysis of transcript levels Quantitative real-time RT–PCR (qRT–PCR) was used to measure transcript levels. RNA sample preparation, reverse transcription and quantitative–PCR were carried out based on the rules that have recently been proposed [23] to ensure reproducible and accurate measurements. Extraction of total RNA samples from appropriate plant materials and RT–PCR conditions have been described previously [24] . The RNA samples were pretreated extensively with an RNAse-free DNAse to eliminate any contaminating genomic DNA before use. qRT–PCR was carried out in 96-well blocks using an Applied Biosystems 7500 Real-Time PCR System (Applied Biosystems) using the SYBR Green I master mix in a volume of 25 μl. The PCR primers were designed using the Primer Express Software installed into the System and listed in Supplementary Table S2 . The two-step thermal cycling profile used was 15 s at 94 °C and 1 min at 68 °C. An eIF4A gene (At3g13920) was included in the reactions as an internal control for normalizing the variations in cDNA amounts used [25] . All qRT–PCR reactions were carried out in biological triplicates using RNA samples extracted from three independent plant materials grown under identical growth conditions. The comparative ΔΔ C T method was used to evaluate relative quantities of each amplified product in the samples. The threshold cycle ( C T ) was automatically determined for each reaction by the System set with default parameters. The specificity of the PCR reactions was determined by melt curve analysis of the amplified products using the standard method installed in the System. Subcellular localization of IDD14 proteins For detection by fluorescence microscopy, the red fluorescent protein (RFP)- and green fluorescent protein (GFP)-coding sequences were fused in-frame to the 3′ ends of the IDD14α and IDD14β sequences, respectively, and the fusions were subcloned into the p326-RFP vector for RFP fusion and the pB7FWG2 vector for GFP fusion. The expression constructs were transformed into Arabidopsis protoplasts by polyethylene glycol-calcium transfection [26] . The subcellular distribution of the IDD14 proteins was visualized by differential interference contrast (DIC) microscopy and fluorescence microscopy. The GFP and RFP fusion proteins were excited at 488 and 568 nm, and the green and red fluorescence signals were filtered with HQ515/30 and HQ600/50 emission filters, respectively. The auto-fluorescence of chlorophylls was excited at 568 nm and emitted with the E600LP filter. The merged signals were obtained using a Confocal Assistant 4.02 (Todd Clark Brelje, Freeware). Yeast two-hybrid assays Yeast two-hybrid assays were performed using the BD Matchmaker system (Clontech). The pGADT7 vector was used for GAL4 AD (activation domain), and the pGBKT7 vector was used for GAL4 BD (DNA-binding domain). The yeast strain AH109 (Leu-, Trp-, Ade-, His-), which has chromosomally integrated reporter genes lacZ and HIS under the control of the GAL1 promoter, was used for transformation. The PCR products were digested with Nde I and Eco RI and subcloned into the pGBKT7 and pGADT7 vectors. Transformation of the AH109 cells was performed according to the manufacturer's instructions. Colonies obtained were streaked on a medium without His, Ade, Leu and Trp. To confirm the results, β-Gal assays were carried out according to the system procedure. For colony filter-lift assays, yeast cells carrying different combinations of plasmids were grown on –LW plate and transferred to a Whatman no. 5 paper filter. Cells were permeabilized by freeze-thaw treatment of the filters. The filters carrying the cells were then placed over filters presoaked with Z-buffer-X-Gal solution according to the protocol of the Matchmaker system. The pBridge vector (Clontech) was used for yeast three-hybrid screening. The IDD14α cDNA was amplified by RT–PCR, and the PCR product was digested with Eco RI and Sal I and subcloned into the pBridge vector, resulting in the BD-IDD14α construct. The IDD14β cDNA was subcloned into the Not I-digested pBridge vector so that its expression was controlled by the pMET25 promoter. The expression constructs (BD-IDD14α and pMET25-IDD14β in the pBridge vector and AD-IDD14α in the pGADT7 vector) were cotransformed into the AH109 cells. The colonies were streaked on media without Leu, Trp and His supplemented with or without methionine. In vitro pull-down assays Recombinant MBP and MBP-IDD14α proteins were produced in Escherichia coli BL21-CodonPlus (DE3)-RIL strains (Stratagene) and purified as follows. One-tenth volume of precultured cells (5 ml) was added to 500 ml of fresh Luria-Bertani medium and cultured at 37 °C until OD 600 reached 0.3–0.6. Protein production was induced by adding isopropyl-β- D -thiogalactopyranoside at a final concentration of 0.5 mM and shaking at 37 °C for 5 h. Cells were collected and resuspended in buffer A (25 mM HEPES, pH 7.5, 20% glycerol, 1 mM dithiothreitol, 100 mM NaCl, 0.2 mM EDTA with protease inhibitor cocktail (Sigma-Aldrich), and 1 mM phenylmethyl sulphonyl fluoride). The cells were lysed using a French press (8500 p.s.i. ; one time). The lysates were sonicated for 30 s twice and centrifuged at 20,000 g for 20 min. The supernatants were stored at −80 °C until use. The IDD14α and IDD14β cDNAs were amplified by RT–PCR and were subcloned into the pGADT7 vector. The IDD14α and IDD14β polypeptides were labelled with 35 S-Met using the TNT-coupled reticulocyte lysate system (Promega). The MBP or MBP-IDD14α proteins were mixed with amylose resin (Sigma-Aldrich) and agitated for 15 min at room temperature. The beads were then washed three times with 1× PBS buffer and one time with buffer A. Five μl of the 35 S-labelled proteins was added and incubated for 2 h at 4 °C. The beads were then washed five times with buffer A. The bound proteins were eluted with 1× SDS-loading buffer by boiling for 5 min at 100 °C and subject to SDS–polyacrylamide gel electrophoresis (PAGE) and autoradiography. Interactions between IDD14α and IDD14β were also examined by immunoprecipitation assays. The IDD14α-MYC and IDD14β-MYC gene fusions, in which a MYC-coding sequence was fused in-frame to the 3′ ends of the IDD14α and IDD14β genes, were expressed transiently in leaf cells of N. benthamiana as described previously [4] . The recombinant MBP-IDD14α fusion protein was prepared in E. coli cells. Total proteins were extracted from the N. benthamiana leaf cells and mixed with the recombinant MBP-IDD14α protein using extraction buffer (50 mM HEPES, pH 7.9, 20% glycerol, 1 mM dithiothreitol, 100 mM NaCl and 0.2 mM EDTA) containing a protease inhibitor cocktail (Sigma-Aldrich). After incubation at 4 °C for 6 h, the mixtures were immunoprecipitated using amylose resin. The beads were washed four times with fresh extraction buffer supplemented with 0.1% Triton X-100, and the bound proteins were eluted with 1× SDS–PAGE loading buffer. The eluted proteins were subject to SDS–PAGE, and the IDD14α-MYC and IDD14β-MYC fusion proteins were detected by western blot analysis using an anti-MYC antibody. Bimolecular fluorescence complementation assays BiFC assays were carried out by co-transfection of the IDD14α-nYFP and IDD14β-cYFP vectors or vice versa into the Arabidopsis mesophyll protoplasts as described previously [26] . Sixteen hours after transfection, reconstitution of yellow fluorescent protein (YFP) fluorescence was observed using a confocal microscope with the following YFP filter set up: excitation 515 nm, 458/514 dichroic and emission 560–615 BP filter. Measurement of starch contents For individual assays, ∼ 0.5 g of aerial plant parts was used to measure contents of soluble sugars using the Sucrose/ D -Glucose Assay kit or the Starch Assay kit, according to the manufacturer's protocols (Megazyme). After grinding plant materials in liquid nitrogen, soluble sugars were extracted two times with 80% ethanol at 70 °C, and fractions were collected. They were then centrifuged at 12,000 g for 10 min. Ethanol was evaporated from the supernatant using a vacuum evaporator, and the solution volume was adjusted to 400 μl by adding triple-distilled water to measure sugar contents. The insoluble pellets were used to measure starch contents. Chromatin immunoprecipitation assays A MYC-coding sequence was fused in-frame to the 3′ ends of the IDD14α and IDD14β genes, and the fusions were subcloned under the control of the CaMV 35S promoter. The expression construct was transformed into Arabidopsis plants. Three-week-old 35S: IDD14α-MYC and 35S: IDD14β-MYC transgenic plants grown on 1/2× Murashige and Skoog agar plates were used for extraction of total cellular extracts. Processing of plant materials and qRT–PCR were carried out as described previously [27] . The qRT–PCR primers used are listed in Supplementary Table S3 . Transcriptional activation activity assays For transient expression assays in Arabidopsis protoplasts, several reporter and effector plasmids were constructed. The reporter plasmid contains four copies of the GAL4 upstream activation sequence and the β-glucuronidase ( GUS ) gene. To construct the p35S: IDD14 effector plasmids, the IDD14α and IDD14β genes were fused to the GAL4 DNA-binding domain and inserted into an expression vector containing the CaMV 35S promoter. The reporter and effector plasmids were cotransformed into Arabidopsis protoplasts by a polyethylene glycol-mediated transformation method. The GUS activities were measured by the fluorometric method as described previously [28] . A CaMV 35S promoter-luciferase (LUC) construct was also cotransformed as an internal control. The luciferase assay was carried using the Luciferase Assay System kit (Promega). How to cite this article: Seo, P. J. et al . Two splice variants of the IDD14 transcription factor competitively form nonfunctional heterodimers, which may regulate starch metabolism. Nat. Commun. 2:303 doi: 10.1038/ncomms1303 (2011).